Unstacked double-layer templated graphene for high-rate lithium–sulphur batteries Preventing the stacking of graphene is essential to exploiting its full potential in energy-storage applications. The introduction of spacers into graphene layers always results in a change in the intrinsic properties of graphene and/or induces complexity at the interfaces. Here we show the synthesis of an intrinsically unstacked double-layer templated graphene via template-directed chemical vapour deposition. The as-obtained graphene is composed of two unstacked graphene layers separated by a large amount of mesosized protuberances and can be used for high-power lithium–sulphur batteries with excellent high-rate performance. Even after 1,000 cycles, high reversible capacities of ca . 530 mA h g −1 and 380 mA h g −1 are retained at 5 C and 10 C, respectively. This type of double-layer graphene is expected to be an important platform that will enable the investigation of stabilized three-dimensional topological porous systems and demonstrate the potential of unstacked graphene materials for advanced energy storage, environmental protection, nanocomposite and healthcare applications. Graphene is a promising functional material for a variety of applications because of its extraordinary electronic and mechanical properties [1] . In response to urgent energy and environmental issues, the applications of graphene in energy storage and conversion have been widely investigated [2] , [3] , [4] , [5] . However, the huge surface area and strong π–π interactions between graphene layers lead to their facile stacking, with an interlayer distance of ca . 0.334 nm; this stacking results in a much smaller surface area of the as-obtained graphene and poor energy-storage performance. To amplify the intrinsic properties of graphene, its stacking needs to be effectively prevented. Numerous novel approaches have been explored to inhibit the stacking of graphene. Most of them are based on the introduction of spacers such as metal oxides [6] , conducting polymers [7] , [8] , carbon black [9] , or carbon nanotubes (CNTs) [10] , [11] , [12] into the interlayer spaces. However, such hybridization processes always result in changes in the intrinsic properties of graphene and/or induce poor interfaces. In addition, the graphene involved in these reports is typically chemically-derived from the liquid exfoliation and reduction of graphene oxide. Chemically-derived graphene materials usually possess severe structural defects and poor electrical conductivity [13] , [14] . Chemical activation and integration methods have been developed to facilitate the mesoporous and hierarchical porous structure of graphene materials to improve their surface area and, thus, their electrochemical properties [15] , [16] , [17] . However, the stacking of graphene is still not easily prevented, and the conductivity of chemically-derived graphene materials decreases as more defects are introduced. The existence of curvatures and wrinkles on graphene can prevent the stacking of graphene to a certain extent and make the single-layer graphene thermally stable, but their presence is not sufficient to fully prevent the stacking [1] . We then come to the idea that the stacking of the as-obtained graphene would be very difficult if every individual graphene-layer building block contains a large amount of protuberances. Such intrinsically unstacked graphene is expected to possess a large surface area, a controllable three-dimensional (3D) nanostructure and conductive scaffolds, as well as robust frameworks formed by sp 2 carbon–carbon bonding. This spacer-free graphene is expected to provide abundant interfaces between the conductive frameworks and ionic channels for electrochemical energy storage. The synthesis of large-sized graphene via the annealing of SiC and chemical vapour deposition (CVD) on metal substrates can lead to high-quality graphene with improved electrical conductivity. This method is also effective for the growth of single-layer graphene through adjustment of the growth parameters [18] . Furthermore, the direct growth method also allows the templated growth of graphene with an anticipated morphology. In general, the morphology of highly electrically conductive graphene grown by CVD depends on the morphology of the template catalysts [19] , [20] , [21] , [22] . On the basis of the fact that metal oxides actively decompose the carbon source and deposit single-layer graphene due to the exposed oxygen atoms on their surface, we explored the idea of epitaxial growth of unstacked graphene with intrinsic protuberances on a mesoporous metal oxide nanosheet by template-directed CVD. As illustrated in Fig. 1 , mesoporous nanoflakes are employed as the template. The graphene layers are deposited onto the mesoporous template and cast into its mesoporous structure, where the carbon atoms deposited in the mesopores form the graphene protuberances and act as spacers to prevent the stacking of the graphene layers deposited on both sides of the mesoporous flakes. Consequently, unstacked double-layer template graphene (DTG) composed of two graphene layers with a large quantity of protuberances can be recovered after the removal of the mesoporous flakes. Because of the mesoporous structure, high surface area and high electrical conductivity of the CVD-grown graphene building block, the DTG is expected to act as an effective electrode material for high-power lithium–sulphur (Li–S) batteries. 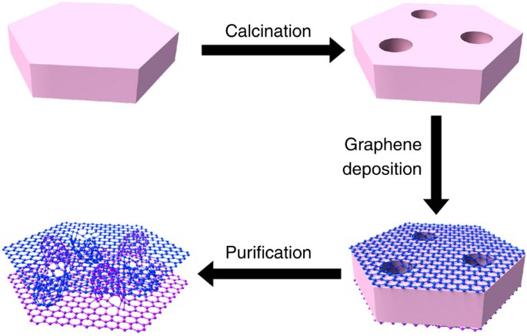Figure 1: Scheme for the synthesis of unstacked DTG. A mesoporous metal oxide derived from the calcination of layered double hydroxide nanoflakes was used as a template to cast DTG. The template was removed by etching, whereas the DTG was unstacked due to the protuberances extending from the graphene sheets. Figure 1: Scheme for the synthesis of unstacked DTG. A mesoporous metal oxide derived from the calcination of layered double hydroxide nanoflakes was used as a template to cast DTG. The template was removed by etching, whereas the DTG was unstacked due to the protuberances extending from the graphene sheets. Full size image Deposition of the DTG onto metal oxide flakes MgAl-layered double oxide (LDO) flakes obtained by the calcination of MgAl-layered double hydroxides (LDHs) were adopted as mesoporous catalysts for the templated growth of DTG. The LDHs are an anionic hydrotalcite-like material composed of positively charged layers and charge-balancing interlayer anions [23] , [24] . The as-prepared MgAl LDHs were hexagonal flakes with a uniform lateral size of ca . 2 μm and a thickness of ca . 10 nm ( Fig. 2a ). A powder X-ray diffraction (XRD) pattern revealed that the as-synthesized MgAl LDH flakes were well crystallized, with lattice parameters of a =0.304 nm and c =2.238 nm ( Fig. 2b ). In situ XRD analysis was performed to investigate the topological evolution of the MgAl LDHs during the calcination, which involved several steps: the removal of interlayer H 2 O molecules (180–260 °C), dehydration caused by the decomposition of OH − in the positively charged LDH layers (260–380 °C), decarbonization caused by the decomposition of interlayer CO 3 2− (>380 °C) and the formation of a MgAl 2 O 4 spinel phase (>780 °C) ( Supplementary Fig. 1 ). After calcination at 950 °C for 30 min, the hydrotalcite-like structure of the MgAl LDHs was completely destroyed, leaving MgO and MgAl 2 O 4 as the main components for the resulting MgAl LDOs ( Fig. 2b ). However, the plate-like morphology and layered structure of the LDH flakes were preserved ( Supplementary Fig. 2a,b ). In addition, numerous closed mesopores were observed in the transmission electron microscopy (TEM) images of the MgAl LDO flakes ( Supplementary Fig. 2c ). These closed mesopores are due to the Kirkendall diffusion of Mg 2+ during the transformation of octahedral Mg–O into tetrahedral Mg–O via dehydration of the interface –OH groups. The mesoporous structure of the MgAl LDOs was further confirmed by their N 2 adsorption behaviour and by their as-calculated pore size distribution ( Supplementary Fig. 3 ). Notably, the MgAl LDOs exhibited a monocrystal-like structure rather than randomly mixed metal oxides and spinels, as indicated by the clear hexagonal diffraction pattern in the selected area electron diffraction pattern of the LDO flakes ( Supplementary Fig. 2d ). Such LDO flakes with an oxygen-terminated surface can catalyse the decomposition of a carbon source for the uniform deposition of graphene on their exposed surfaces. After the CVD of CH 4 onto the MgAl LDO flakes, a diffraction peak was detected at 13.3° in the XRD pattern of the as-obtained MgAl LDO/graphene composites; this peak was ascribed to the contribution of the interspace between the deposited carbon layers and the surface of the LDO flakes. No obvious difference between the morphology of the LDO/graphene composites and that of the LDO flakes ( Fig. 2c ) was evident in the TEM images. However, deposited graphene layers can be clearly observed on the surface of the MgAl LDO flakes and in their mesopores in the high-resolution TEM images ( Fig. 2d,e ). 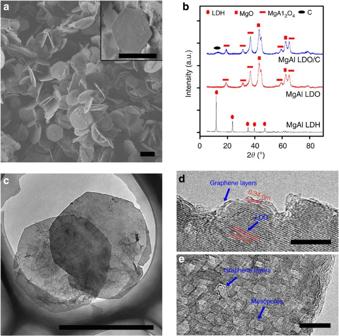Figure 2: Nanostructure of the templates for unstacked DTG deposition. (a) Scanning electron microscope image and (b) XRD patterns of MgAl LDH precursors and the products after the calcination and carbon deposition. (c) TEM images of the calcined MgAl LDHs with a well-preserved flake morphology after being treated at a very high temperature of 950 °C. (d,e) High-resolution TEM images of graphene nanosheets cast onto the LDO flakes. The scale bar in (a,c) equals 2 μm. The scale bar in (d,e) equals 10 nm. Figure 2: Nanostructure of the templates for unstacked DTG deposition. ( a ) Scanning electron microscope image and ( b ) XRD patterns of MgAl LDH precursors and the products after the calcination and carbon deposition. ( c ) TEM images of the calcined MgAl LDHs with a well-preserved flake morphology after being treated at a very high temperature of 950 °C. ( d , e ) High-resolution TEM images of graphene nanosheets cast onto the LDO flakes. The scale bar in ( a , c ) equals 2 μm. The scale bar in ( d , e ) equals 10 nm. Full size image Morphology and structural analysis of the DTG Both the scanning He-ion microscopy and the TEM images indicate that the as-obtained graphene after the removal of LDOs from the LDO/graphene composites exhibit a hexagonal morphology and size similar to those of the original LDO flakes ( Fig. 3a and Supplementary Fig. 4a ). The porous-like hexagonal graphene was uniformly cast onto the LDO flakes, and pores that appeared as circular graphene layers with a size of several nanometres were located on the as-obtained graphene ( Fig. 3b ). No graphene layer was observed on one side of the pores in most cases; however, two graphene layers were observed on the other side of the pores on the as-obtained single-layer graphene sheet, as indicated by the black arrow in Fig. 3c . This result indicates that the pores on the graphene did not result from the cavities; they were rather constructed by a very small graphene protuberance with a structure similar to an ultra-short CNT on the graphene [11] . The atomic force microscopy (AFM) image shown in Supplementary Fig. 4b reveals that the as-obtained DTG exhibits a thickness of ca . 10 nm, although only a few layers (<3) of graphene was deposited on both sides of the LDO flakes, which indicates that the interspace distance between the up/down layers of DTG is up to several nanometres and the stacking of the two graphene layers of DTG is effectively prevented. The high-resolution AFM image of the DTG samples after a strong sonication (300 W) for 2 h clearly illustrated the large amount of protuberances on the surface of the graphene, which was considered to be the morphology of the single graphene building blocks of the DTG ( Supplementary Fig. 4c ). Therefore, we concluded that the presence of the protuberances successfully prevented the stacking of the two graphene layers deposited uniformly on both sides of the LDO flakes after the templates were removed. The as-obtained DTG exhibited a lamellar box-like structure composed of two unstacked graphene layers separated by a large quantity of protuberances ( Fig. 1 ). Statistical results from numerous TEM images showed that the protuberances were uniformly distributed over the DTG, with a density of ca . 5.8 × 10 14 m −2 and a size between 2 and 8 nm ( Supplementary Fig. 5 ). Notably, the presence of such protuberances on the surface of graphene can weaken the π–π interactions between graphene layers and thus prevent the stacking of neighbouring DTG to a certain extent. This observation was confirmed by the scanning electron microscope images in Supplementary Fig. 6a–c showing the loose stacking of a large amount of DTG and by the fact that individual DTG flakes were easily obtained by a simple sonication in ethanol ( Fig. 3a and Supplementary Fig. 4a ). The formation of graphene protuberances is attributed to the graphene being cast on the inner surface of the mesopores of the LDO templates. Because of their strong interaction, the protuberances prefer to lie down on the graphene layer ( Fig. 3c ). Notably, the structure of the MgAl LDO flakes is quite different from that of MgO sheets obtained by calcination of Mg(OH) 2 sheets [25] , [26] , which can be considered an aggregate of MgO nanocrystals. Herein, the uniform and monocrystal-like structure of LDOs decorated by a large quantity of mesopores gives rise to an uninterrupted and uniform unstacked graphene layer with protuberances rather than an aggregate of graphene nanocages ( Fig. 3b–d ), which ensures that the electrical conductivity of the as-obtained DTG will be substantially improved. 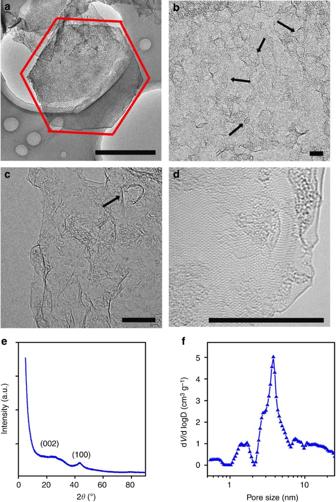Figure 3: Nanostructure of the unstacked DTG. (a,b) TEM images of the cast DTG flakes. (c,d) High-resolution TEM images of DTG with protuberances extending from the graphene sheets and the graphene layer for DTG; (e) XRD pattern and (f) pore size distribution of the DTG. The scale bar in (a) and (b–d) equals 1 μm and 10 nm, respectively. Figure 3: Nanostructure of the unstacked DTG. ( a , b ) TEM images of the cast DTG flakes. ( c , d ) High-resolution TEM images of DTG with protuberances extending from the graphene sheets and the graphene layer for DTG; ( e ) XRD pattern and ( f ) pore size distribution of the DTG. The scale bar in ( a ) and ( b – d ) equals 1 μm and 10 nm, respectively. Full size image Characterization of the DTG sample by XRD revealed that the (002) peak of the DTG has a markedly low intensity and is dramatically broad ( Fig. 3e ), which is attributed to the fact that the DTG is composed of predominantly single-layer graphene. The large increase in the region below 10° and the broad peak in the low-angle XRD pattern indicate the enlarged d-space of the as-obtained DTG and the presence of a high density of mesosized protuberances ( Fig. 3e and Supplementary Fig. 7 ). The specific surface area (SSA) and pore size characterization of the DTG were performed by N 2 adsorption/desorption experiments ( Fig. 3f and Supplementary Fig. 8 ). The DTG shows a high SSA of 1,628 m 2 g −1 , as calculated via the Brunauer–Emmett–Teller (BET) method. The pore size distribution of the sample was calculated on the basis of the density functional theory model ( Fig. 3e ). A large quantity of mesopores with sizes of 2–7 nm were available for the DTG. The DTG pore size distribution is very similar to that of the LDOs; however, the DTG exhibits a much larger pore volume. The total pore volumes of the DTG and LDOs are 2.0 and 0.18 cm 3 g −1 , respectively. The enlarged pore volume of DTG compared with that of the LDO flakes is considered to arise from the interlayer space of the two graphene layers deposited on both sides of the LDO flakes. The roots of the protuberances covalently bond with the graphene layers and the tips of the protuberances pillar the opposite graphene layer. The interlayer space of the DTG constructs the main mesoporous structure of the as-prepared DTG. The mesoscale interlayer space of DTG, as opposed to the microporous structure of graphite, further demonstrates the unstacked feature of DTG, which is attributed to the presence of the protuberances. Thermogravimetric analysis (TGA) under an oxygen atmosphere revealed that the DTG exhibits good thermal stability, as indicated by a sharp weight loss peak at ~600 °C ( Supplementary Fig. 9a ). The Raman spectrum of the DTG indicates a high defect density, which might be associated with the presence of a large quantity of five- and six-membered carbon rings for the covalent connections between the protuberances and the graphene layers ( Supplementary Fig. 9b ). In addition, the X-ray photoelectron spectroscopy (XPS) results ( Supplementary Fig. 10 ) revealed that the surface of the DTG contains very few O ( ca . 0.9 at.%) atoms and that the C atoms are mainly sp 2 hybridized. Construction of the DTG/S nanocomposites The expected high electrical conductivity derived from the CVD-grown graphene and its mesoporous structure make the as-fabricated DTG a promising cathode material for Li–S batteries, which are a power source with the advantages of low cost, low toxicity, abundant raw materials and an ultra-high theoretical energy density of 2,567 W h kg −1 (more than five times that of conventional lithium-ion batteries) [5] , [27] , [28] , [29] . To evaluate their electrochemical performance, we fabricated the DTG/S nanocomposites using a melt-diffusion strategy and used the nanocomposites as the cathode materials in Li–S cells. The incorporation of sulphur into the DTG induced no obvious changes in their morphology ( Fig. 4a , Supplementary Fig. 6d–f ). No bulk sulphur particles were detected on the external surface of the DTG. The TEM images in Fig. 4a,b indicate that the sulphur is homogeneously dispersed in the DTG, and the high-resolution TEM image in Fig. 4c reveals that the sulphur nanoparticles can also be incorporated in the mesosized protuberances on the DTG. Therefore, the sulphur was homogeneously dispersed in the DTG/S nanocomposites ( Fig. 4d–f ). A high sulphur loading of ca . 64 wt% was determined ( Fig. 4g ). The weight loss that resulted from the volatilization of sulphur in the DTG/S nanocomposites occurred at 210–430 °C, which is a higher temperature than that at which pure sulphur volatilizes (160–270 °C), indicating the strong interaction between the DTG and the sulphur and the effective trapping of sulphur in the porous structure of the DTG. 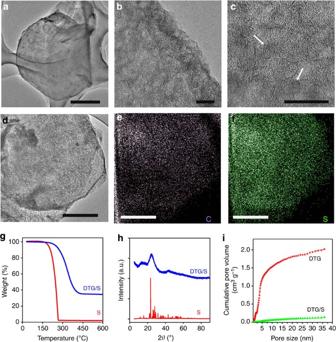Figure 4: The unstacked DTG-supported sulphur cathode. (a,b) TEM and (c) high-resolution TEM images of the DTG/S cathode; (d) TEM and (e,f) energy-dispersive X-ray spectroscopy maps of C and S in the DTG/S cathode. (g) TGA trace, (h) XRD pattern and (i) cumulative pore volume of the DTG/S cathode. Ultrafine sulphur clusters were uniformly distributed on the DTG. The scale bar in (a), (b,c) and (d-f) equals 1, 20 and 0.5 μm, respectively. Figure 4h and Supplementary Fig. 7 present the XRD patterns for elemental sulphur and the as-prepared DTG/S nanocomposites. No clear characteristic peak of sulphur was present in the XRD pattern of DTG/S, further indicating the good distribution of incorporated sulphur. Most of the mesopores of the DTG are filled with sulphur, as indicated by the fact that the pore volume of the DTG after the incorporation of sulphur decreased markedly from 2.0 to 0.13 cm 3 g −1 ( Fig. 4i and Supplementary Fig. 11 ). Sulphur is incorporated not only in the mesoscale protuberances of DTG but also in the interlayer space, which can accommodate sulphur and reduce the dissolution of the corresponding Li polysulphides into the electrolyte much more effectively. The SSA calculated by the BET method decreased from 1,628 m 2 g −1 for DTG to 39 m 2 g −1 for the DTG/S nanocomposite, indicating effective contact between the graphene layers and the accommodated sulphur, which is of paramount importance for rapid electron transport. Figure 4: The unstacked DTG-supported sulphur cathode. ( a , b ) TEM and ( c ) high-resolution TEM images of the DTG/S cathode; ( d ) TEM and ( e , f ) energy-dispersive X-ray spectroscopy maps of C and S in the DTG/S cathode. ( g ) TGA trace, ( h ) XRD pattern and ( i ) cumulative pore volume of the DTG/S cathode. Ultrafine sulphur clusters were uniformly distributed on the DTG. The scale bar in ( a ), ( b , c ) and ( d - f ) equals 1, 20 and 0.5 μm, respectively. Full size image Electrochemical performance of the DTG/S cathode materials Coil cells were fabricated to evaluate the electrochemical Li storage capability of the DTG/S cathode material using Li foil as the anode. 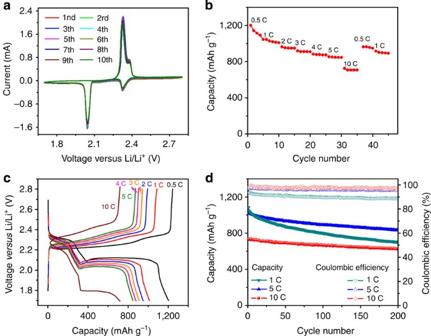Figure 5: Performance of a Li–S battery with a DTG/S cathode. (a) CV profile of the DTG/S cathode. (b) Rate performance of the DTG/S cathode. (c) Charge–discharge curves of the DTG/S cathode. (d) Long cycle performance of the DTG/S cathode at 1.0, 5.0 and 10.0 C. Figure 5 shows the electrochemical performance of the DTG/S nanocomposite. The cyclic voltammogram (CV) profile conducted at a scan rate of 0.1 mV s −1 is shown in Fig. 5a . Two main peaks are observed during the cathodic scan, indicating that the reduction process occurs in two stages. According to the reported mechanisms for the reduction and oxidation of sulphur during the charge/discharge process, the first peak at ~2.32 V corresponds to the reduction of elemental sulphur to higher-order Li polysulphides (Li 2 S n , 4≤ n <8). The second peak at ~2.04 V corresponds to the further reduction of the higher-order Li polysulphides to Li 2 S 2 and, eventually, to Li 2 S. The oxidation process of the cathode also occurs in two stages. The first oxidation peak at ~2.33 V is associated with the formation of Li 2 S n ( n >2), which is oxidized to elemental sulphur at ~2.38 V. Over 10 cycles, both the CV peak positions and the peak currents change only slightly, indicating that the DTG effectively prevents sulphur from dissolving into the electrolyte. At a current rate of 0.5 C, a reversible capacity of ~1,200 mA h g −1 was achieved ( Fig. 5b ). The rate capability of the DTG/S nanocomposites gradually decreased with increasing current rate, but the nanocomposites exhibited much improved cycling stability. A reversible high and stable capacity of 857 mA h g −1 was retained even at a very high current rate of 5.0 C, exhibiting only a 16.0% decrease compared with that at 1.0 C. At the maximum investigated discharge rate of 10 C, the capacity of the DTG/S nanocomposites was still as high as 713 mA h g −1 . After the cells were charged at a rather high rate of 10.0 C, the capacities recovered to 961 mA h g −1 and 901 mA h g −1 at 0.5 C and 1.0 C, respectively. Figure 5c reports typical discharge/charge voltage profiles of the electrodes at different current rates. All of the discharge curves contain two plateaus that correspond to the peaks in the CV profiles. The cycle-life behaviour of the DTG/S nanocomposites is shown in Fig. 5d . At a current rate of 1.0 C, an initial capacity of 1,084 mA h g −1 was achieved. This capacity decreased to 800 mA h g −1 after 100 cycles, which represents a capacity fade of 26.2%, and to 701 mA h g −1 after 200 cycles, which represents a 35.4% fade. When the current rate was increased to 5.0 C, an improved cycle stability was achieved, and the capacity decreased from 1,034 to 832 mA h g −1 , which represents a decay of 19.5%, after 200 cycles. In addition, the coulombic efficiency of the DTG/S electrode was improved from ~90% at 1 C to ~96% at 5.0 C. These results indicate that the shuttling effect was effectively prevented with increasing current rate because of a much faster charge/discharge process [30] . When the current rate was further increased to 10.0 C, both the cycling stability and the coulombic efficiency were further improved. An initial capacity of 734 mA h g −1 was achieved, and it decreased to 628 mA h g −1 after 200 cycles, indicating a stable efficiency of ca . 98%. Even after 1,000 cycles, high reversible capacities of ca . 530 mA h g −1 and 380 mA h g −1 were still retained at 5.0 C and 10.0 C, respectively ( Supplementary Fig. 12 ). Figure 5: Performance of a Li–S battery with a DTG/S cathode. ( a ) CV profile of the DTG/S cathode. ( b ) Rate performance of the DTG/S cathode. ( c ) Charge–discharge curves of the DTG/S cathode. ( d ) Long cycle performance of the DTG/S cathode at 1.0, 5.0 and 10.0 C. Full size image The excellent high-rate performance of the DTG/S nanocomposites is attributed to the extraordinary electrical conductivity and unique mesoporous structure of the DTG. A high electrical conductivity of 438 S cm −1 was determined using the four-probe technique on a DTG disk with a diameter of 13.0 mm and a thickness of ca . 10 μm, which was prepared by compression at 5.0 MPa. After the infiltration of sulphur into the DTG, the electrical conductivity of the DTG/S composites measured by the same method was reduced to 107 S cm −1 , which can be ascribed to the unavoidable coverage of the outer surface of the DTG with some amount of elemental sulphur. Electrochemical impedance spectroscopy of the cathode was also performed to further demonstrate the good electrical conductivity of the DTG. Charge transfer resistances of 13.4 Ω and 13.1 Ω were determined for the DTG/S cathode before and after the CV test, respectively ( Supplementary Fig. 13 and Supplementary Table 1 ), which were much lower than those observed when multi-walled CNTs, single-walled CNTs, graphene and polyacrylonitrile-coated graphene were used as the cathode materials [31] , [32] , [33] , [34] . In addition to its excellent electrical conductivity, DTG’s unique porous structure allows the effective storage of sulphur in the mesosized lamellar interlayer space, which gives rise to an efficient connection between sulphur and graphene and prevents the diffusion of polysulphides into the electrolyte. Consequently, an excellent high-rate performance of the DTG/S cathode with a high capacity and good stability is achieved. In summary, DTG composed of two unstacked graphene layers separated by a large quantity of protuberances was synthesized using template-directed CVD of graphene layers on mesoporous LDH-derived flakes and served as the cathode material for Li–S batteries after the incorporation of sulphur into the mesopores. The high surface area of the DTG provides effective contact between the incorporated sulphur and the graphene layers, and its mesoporous structure encapsulates part of the electrochemically generated Li polysulphide species. The as-fabricated Li–S cells with DTG/S nanocomposites as the cathode and Li foil as the anode exhibited excellent high-rate performance because of the high electronic conductivity of the CVD-grown graphene layers and the effective retention of sulphur in their mesoporous structures. High reversible capacities of 1,034 mA h g −1 and 734 mA h g −1 were achieved at high discharge rates of 5 C and 10 C, respectively. Even after 1,000 cycles, high reversible capacities of ca . 530 and 380 mA h g −1 were retained at 5 and 10 C, with coulombic efficiency constants at ca . 96% and 98%, respectively. The preparation of the unstacked DTG is scalable and serves as a general strategy for the fabrication of a broad class of electrode materials for supercapacitors and lithium-ion, lithium–sulphur and lithium–air batteries. We expect these DTG materials to have potential applications in the areas of environmental protection, nanocomposites, electronic devices and healthcare because of their intrinsic large surface area, extraordinary thermal and electric conductivity, robust 3D scaffold, tunable surface chemistry and biocompatible interface. Because unstacked layered nanostructures are not limited to graphene, we foresee a new branch of chemistry evolving in the stabilization of nanostructures through 3D topological porous systems. Synthesis The MgAl LDHs were prepared using a urea-assisted co-precipitation reaction. Mg(NO 3 ) 2 ·6H 2 O, Al(NO 3 ) 3 ·9H 2 O and urea were dissolved in 250.0 ml of deionized water with [Mg 2+ ]+[Al 3+ ]=0.15 mol l −1 , n (Mg): n (Al)=2:1 and [urea]=3.0 mol l −1 . The as-obtained solution was maintained at 100 °C under continuous magnetic stirring for 12 h in a flask (equipped with a reflux condenser) of 500.0 ml under ambient atmosphere. Then, the prepared suspension was kept at 94 °C for another 12 h without stirring. The as-prepared MgAl LDH flakes were obtained after the product was filtered, washed and freeze dried. The DTG was prepared by CVD with calcined LDHs as the templates. First, MgAl LDH flakes were sprayed uniformly into a quartz boat, which was placed at the centre of a horizontal quartz tube inserted into a furnace, where the sample was under atmospheric pressure. The furnace was subsequently heated to 950 °C and maintained there for 30 min under flowing Ar (200 ml min −1 ). Afterwards, CH 4 (600 ml min −1 ) was introduced into the reactor for the deposition of graphene. The reaction was maintained for 10 min before the furnace was cooled to room temperature under Ar protection. The as-obtained products were purified by sequential alkali (15.0 mol l −1 NaOH aqueous solution) and acid (5.0 mol l −1 HCl aqueous solution) treatments at 80 °C to remove the LDO flakes. The DTG was obtained after the product was filtered, washed and freeze dried. The DTG/S nanocomposite was prepared by a melt-diffusion strategy. Typically, the DTG was first mixed with sulphur powder by milling. The mixture was then placed in a sealed Teflon container at 155 °C for 4 h to incorporate the sulphur into the mesopores of the DTG. Characterization The morphology of the samples were examined using a JSM 7401F (JEOL Ltd.) scanning electron microscope operated at 3.0 kV and a JEM 2010 (JEOL Ltd.) TEM operated at 120.0 kV. Atomically resolved high-resolution TEM observations were conducted on a Titan3 60–300 (FEI Company) microscope operated at 80 kV. The scanning He-ion microscopy images were obtained using a He-ion microscope (Orion NanoFab Imaging system, Carl Zeiss Microscopy) operated at 30 kV. The AFM images were obtained using a SPM-9500J3 apparatus. Energy-dispersive X-ray spectroscopy analyses were performed using a JEM 2010 apparatus in conjunction with the analytical software INCA; the applied accelerating voltage was 120.0 kV. XRD patterns were recorded on a Bruker D8 Advance diffractometer equipped with a Cu-K α radiation source operated at 40.0 kV and 120 mA. Raman spectra were obtained with He–Ne laser excitation at 633 nm using a Horiba Jobin Yvon LabRAM HR800 Raman spectrophotometer. TGA was performed under heating at 10 °C min −1 using a Mettler Toledo TGA/DSC-1 analyzer. The pore size distributions and BET SSAs of the samples were measured by N 2 adsorption at liquid N 2 temperature using an Autosorb-IQ 2 -MP-C system. The XPS spectra were obtained using XPS conducted on an Escalab 250Xi. Electrochemistry Two-electrode cells in the form of standard 2025 coil-type cells were constructed in an Ar-filled glove box to evaluate the electrochemical performance of the DTG as cathode materials for Li–S batteries. The DTG/S cathode slurry was prepared by mixing the DTG/S nanocomposites (90%) and of poly(vinylidene fluoride) binder (10%) in an N -methylpyrrolidone (NMP) solvent dispersant. Positive electrodes were produced by coating the slurry onto aluminium foil and drying at 60 °C for 24 h. The areal density of the electrode was in the range of 0.8–1.1 mg cm −2 . The electrolyte was composed of a 1.0 mol l −1 lithium bis(trifluoromethanesulphonyl)imide solution in 1,3-dioxolane:1,2-dimethoxyethane 1:1 v/v. Approximately 100 μl of electrolyte was used in the fabrication of each Li–S cell. Lithium metal foil was used as the counter electrode and polypropylene membranes from Celgard Inc. were used as separators. The coin cells were tested in galvanostatic mode at various currents within a voltage range of 1.7–2.8 V using a Neware multichannel battery cycler. The CV and electrochemical impedance spectroscopy measurements were performed on a Solartron 1470E electrochemical workstation. A current density of 1,672 mA g −1 (1.0 C) based on the mass of sulphur, which is equivalent to full discharge or charge in 1 h, was applied in both current sweep directions. The capacities were calculated on the basis of the mass of sulphur. How to cite this article: Zhao, M.-Q. et al. Unstacked double-layer templated graphene for high-rate lithium–sulphur batteries. Nat. Commun. 5:3410 doi: 10.1038/ncomms4410 (2014).